Emergent properties of the interferon-signalling network may underlie the success of hepatitis C treatment Current interferon alpha-based treatment of hepatitis C virus (HCV) infection fails to cure a sizeable fraction of patients treated. The cause of this treatment failure remains unknown. Here using mathematical modelling, we predict treatment failure to be a consequence of the emergent properties of the interferon-signalling network. HCV induces bistability in the network, creating a new steady state where it can persist. Cells that admit the new steady state alone are refractory to interferon. Using a model of viral kinetics, we show that when the fraction of cells refractory to interferon in a patient exceeds a critical value, treatment fails. Direct-acting antivirals that suppress HCV replication can eliminate the new steady state, restoring interferon sensitivity and improving treatment response. Our study thus presents a new conceptual basis of HCV persistence and treatment response, elucidates the origin of the synergy between interferon and direct-acting antivirals, and facilitates rational treatment optimization. Hepatitis C virus (HCV) infection is spread over 130–170 million people worldwide [1] . Pegylated interferon-α (IFN-α), in combination with ribavirin, forms the mainstay of the current treatment for HCV infection. The combination (PR), however, elicits a sustained virological response (SVR) in only about 50% of HCV genotype 1 infected patients treated [2] . Several factors that correlate with treatment response have been identified, including HCV genotype, pre-treatment viral load and single-nucleotide polymorphisms (SNPs) in the IFN-λ locus [3] , [4] . The cause of treatment failure, however, remains poorly established. IFN-α belongs to a family of cytokines produced endogenously in response to viral infection [5] , [6] . Through a complex series of signalling events involving the JAK–STAT pathway, stimulation by IFN results in the expression of several hundred IFN-stimulated genes (ISGs) which together induce an antiviral state in cells and control infection [6] . With HCV, however, a vast majority (~70–80%) of infected individuals are unable to clear the infection spontaneously and become chronically infected [6] , [7] . PR treatment can compensate for suboptimal immune control of infection. ISG expression following the onset of treatment was enhanced substantially over the pre-treatment level in the livers of HCV patients who responded to PR [8] , [9] , [10] . (Ribavirin alone elicits no SVR [11] , but improves response in combination with IFN [12] , suggesting that ribavirin potentiates the anti-HCV activity of IFN [10] , [13] , [14] , [15] .) Surprisingly, however, in the livers of nonresponders to PR treatment, pre-treatment ISG expression was higher than in responders and did not increase significantly following the onset of treatment [8] , [9] , [10] . Non-responsiveness to PR was eliminated in part by the recently approved direct-acting antiviral agents (DAAs) telaprevir and boceprevir, each of which in conjunction with PR yielded SVR rates of over 70% in previously untreated HCV genotype 1 infected patients [2] , [16] . Because telaprevir and boceprevir monotherapy fail owing to the emergence of drug resistance, one hypothesis for the success of the triple combination is that DAAs act on drug sensitive strains whereas PR control resistant strains [17] . Paradoxically, however, although the DAAs alone elicited no SVR, the triple combination induced SVR in 40% of previous null responders to PR, who showed no significant decline in viral levels during PR treatment indicating the near absence of IFN activity [18] , [19] . DAAs thus appear to synergize with IFN and help overcome non-responsiveness to PR. In two recent pioneering studies, poor response following high-pre-treatment ISG expression has been suggested to arise from upregulation, associated with persistent IFN signalling, of immunosuppressive molecules such as interleukin-10 and programmed death-ligand 1 (PD-L1), which leads to T-cell exhaustion and viral persistence [20] , [21] . These studies mark a breakthrough in our understanding of chronic viral infections and recommend, counter intuitively, suppression of IFN signalling to avert T-cell exhaustion and elicit control of chronic infection. Two key questions, however, remain unanswered. When does HCV infection lead to high (pre-treatment) ISG expression and therefore poor-treatment response? How, despite high-exogenous IFN addition, which would ensure continued immunosuppression following the onset of treatment, do DAAs improve treatment response in combination with PR? Mechanisms in addition to IFN-associated immunosuppression thus appear to contribute to HCV persistence and treatment response. Previous studies have identified several mechanisms by which HCV evades IFN activity: HCV can suppress endogenous IFN production, inhibit ISG expression by interfering with the JAK–STAT pathway, induce a block in the translation of ISG mRNA, and/or inhibit ISG effector functions [6] , [22] . At the same time, key ISGs involved in the control of HCV have been identified and in some cases their mode of action elucidated [23] , [24] , [25] , [26] , [27] . These specific interactions between HCV and components of the IFN network have unravelled the many fronts of the battle between HCV and our innate immune system. The outcome of this battle, however, has been difficult to predict: the specific interactions prove inadequate for distinguishing between nonresponders and responders to PR or explaining the observed synergy between DAAs and PR, precluding rational strategies for improving treatment response. In the present study, we explore the possibility that responsiveness to IFN is not a consequence of specific molecular interactions between individual components of the IFN system and HCV alone, but of emergent, systems-level properties of the IFN signalling network interacting with HCV. The IFN network is designed to suppress HCV upon stimulation. HCV, on the other hand, interferes with IFN signalling and compromises its effector functions. Non-responsiveness to IFN may thus be a manifestation of the state to which the IFN system is driven as a consequence of these competing interactions. Further, although DAAs directly target viral (or host) proteins, their action may, at the systems level, weaken the influence of HCV on the IFN network and drive the system to an alternative, responsive state. To test this hypothesis, we construct a mathematical model of the IFN signalling network in the presence of HCV and elucidate its systems-level properties. We find intriguingly that HCV induces bistability in the network, causing the emergence of a new steady state where HCV persists. Accounting for this bistability, we develop a mathematical model of viral kinetics and deduce a criterion for treatment response. Finally, we find that DAAs can eliminate this bistability and improve treatment response. Model of the IFN signalling network in the presence of HCV We considered the intracellular IFN signalling network in the presence of HCV ( Fig. 1 ). Upon infection, HCV replicates inside the cell producing copies of positive and negative strands of RNA, the latter presumably existing as double-stranded RNA (dsRNA). In the presence of IFN, ISGs are transcribed to produce ISG mRNA. The translation of ISG mRNA yields ISG proteins, which control HCV by inhibiting different steps of the HCV life cycle and/or lowering the stability of HCV RNA [23] , [24] , [25] , [26] , [27] . Of the ninety ISGs expressed in response to IFN (type I) stimulation, seven were recently found to exhibit significant activity against HCV [24] . HCV can evade IFN action by several mechanisms including lowering global translation in the cell via protein kinase R (PKR) [28] . The latter mechanism has been shown in recent in vitro studies to facilitate HCV persistence despite strong IFN treatment [28] , postulated to be the predominant mode of the interference of IFN signalling by HCV in vivo [29] , and may represent a key pathway underlying the resistance of HCV to IFN [30] . We therefore focused here on the HCV-mediated block in the translation of ISG mRNA via PKR. (We also considered other mechanisms of the interference of IFN signalling by HCV and found similar results; see Discussion.) Initiation of translation depends on the abundance of the eIF2α–guanosine triphosphate (GTP) complex. eIF2α–GTP gets hydrolyzed to eIF2α–guanosine diphosphate (GDP) during translation [31] . The recycling of eIF2α–GDP to eIF2α–GTP is mediated by another protein eIF2B [32] . HCV induces PKR dimerization, presumably by the binding of HCV double-stranded RNA to PKR [33] , [34] . PKR dimers undergo autophosphorylation [34] . Phosphorylated PKR catalyzes the phosphorylation of eIF2α–GDP. Phosphorylated eIF2α–GDP does not undergo GDP to GTP exchange and has an increased affinity for eIF2B [31] , [32] . eIF2B is present in low abundance compared with eIF2α [31] . Thus, phosphorylated eIF2α–GDP sequesters eIF2B, which further reduces the eIF2α–GTP level, blocking translation. HCV, however, continues to replicate as its translation is less sensitive to eIF2α–GTP [28] , [35] , [36] , [37] . The HCV–PKR interaction thus contains key elements of the suppression of IFN activity by HCV as well as the control of HCV by IFN, capturing the essence of the battle between HCV and IFN at the systems level. We modelled the network using a system of coupled differential equations ( Supplementary Note 1 ) and elucidated its emergent properties. 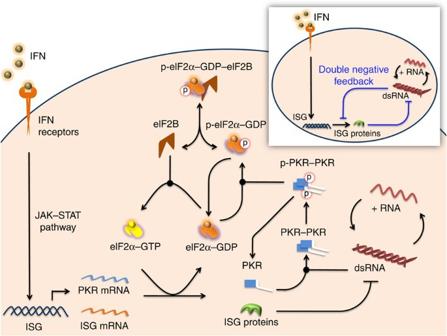Figure 1: Schematic of the IFN signalling network in the presence of HCV. Following exposure to IFN, signalling via the JAK–STAT pathway triggers ISG expression, which lowers the HCV RNA level inside a cell. HCV catalyzes PKR dimerization and autophosphorylation. Phosphorylated PKR phosphorylates eIF2α-GDP, which sequesters eIF2B and lowers translation of ISG mRNA. Inset: schematic of the double-negative feedback in the network owing to the suppression of HCV by ISG proteins and of ISG proteins by HCV. Figure 1: Schematic of the IFN signalling network in the presence of HCV. Following exposure to IFN, signalling via the JAK–STAT pathway triggers ISG expression, which lowers the HCV RNA level inside a cell. HCV catalyzes PKR dimerization and autophosphorylation. Phosphorylated PKR phosphorylates eIF2α-GDP, which sequesters eIF2B and lowers translation of ISG mRNA. Inset: schematic of the double-negative feedback in the network owing to the suppression of HCV by ISG proteins and of ISG proteins by HCV. Full size image Bistability in the IFN signalling network induced by HCV The network exhibits double-negative feedback: ISG proteins control HCV, whereas HCV controls ISG mRNA translation. Double-negative feedback with ultra-sensitivity (nonlinearity) can give rise to bistability [38] , observed in several signalling and transcription networks [38] , [39] , [40] , [41] , [42] . To test the existence of bistability, we identified the steady states of the network as follows. We predicted first the dependence of the steady state ISG protein level on the HCV RNA level (red line in Fig. 2 ). Here the double-stranded HCV RNA level was fixed, thus eliminating the negative feedback of ISG on HCV, and the system solved for steady state. This process was repeated for different values of the double-stranded HCV RNA level. Similarly, we predicted the dependence of the steady state HCV RNA level on the ISG protein level (blue line in Fig. 2 ), by suppressing the negative feedback of HCV on ISG. When both the feedback loops are active, the intersection points Q 1 , Q 2 and Q 3 represent the steady states of the system ( Fig. 2 ). At Q 1 , the HCV RNA level is high and the ISG protein level low, marking HCV persistence, whereas at Q 3 , HCV RNA is absent and the ISG protein level is high, indicating HCV clearance. Q 1 and Q 3 are the two stable steady states of the system. Q 2 , where HCV RNA and ISG protein levels are intermediate, is an unstable steady state, in that small perturbations get amplified and drive the system away from Q 2 . Q 2 , thus acts as a threshold determining which of the two stable steady states the system eventually attains. 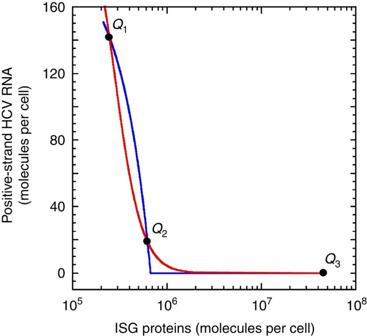Figure 2: HCV-induced bistability in the IFN signalling network. Model predictions of concentration-effect curves showing steady state positive-strand HCV RNA levels for fixed total ISG protein levels (blue line) and total ISG protein levels for fixed double-stranded HCV RNA levels (red line). Both curves are drawn with positive-strand HCV RNA levels on theyaxis and ISG protein levels on thexaxis. The ISG proteins include the seven ISGs, namely, IFIT3, IFITM1, IFITM3, PLSCR1, TRIM14, Viperin and RNase L, identified recently to have anti-HCV activity24(Supplementary Note 1). The intersections of the curves mark the three steady states,Q1,Q2andQ3, of the network. Parameters employed are listed inSupplementary Tables 1–3. Figure 2: HCV-induced bistability in the IFN signalling network. Model predictions of concentration-effect curves showing steady state positive-strand HCV RNA levels for fixed total ISG protein levels (blue line) and total ISG protein levels for fixed double-stranded HCV RNA levels (red line). Both curves are drawn with positive-strand HCV RNA levels on the y axis and ISG protein levels on the x axis. The ISG proteins include the seven ISGs, namely, IFIT3, IFITM1, IFITM3, PLSCR1, TRIM14, Viperin and RNase L, identified recently to have anti-HCV activity [24] ( Supplementary Note 1 ). The intersections of the curves mark the three steady states, Q 1 , Q 2 and Q 3 , of the network. Parameters employed are listed in Supplementary Tables 1–3 . Full size image Bistability in in vitro experiments and model validation Evidence of this threshold and the underlying bistability is found in recent in vitro experiments [28] . In the latter experiments, cells were treated with IFN before or at different times post infection and HCV RNA and ISG protein levels were measured 20 h post IFN treatment [28] . When treated up to 24 h post infection, phosphorylated PKR levels were low, ISG protein levels were high and HCV RNA levels suppressed. When treated ≥48 h post infection, phosphorylated PKR levels were high, ISG protein levels low and HCV RNA levels approached that of IFN untreated cells. Using parameter values obtained independently ( Supplementary Note 2 , Supplementary Tables 1–3 ), our model captured the above observations quantitatively ( Fig. 3a ). According to our model, following infection, the HCV RNA level gradually increases inside cells ( Supplementary Fig. 1A ); endogenous IFN production is not expected in the in vitro cell-culture infection system [43] . If IFN is added when the HCV RNA level is below the threshold corresponding to Q 2 , the system drops to Q 3 , where HCV is controlled. In contrast, if IFN is added after the HCV RNA level crosses the threshold, the system reaches Q 1 , where HCV persists. The switch in the response of the system based on the time of IFN addition is thus a signature of bistability. Indeed, silencing PKR, which suppresses one of the feedback loops, eliminated this signature in the experiments and in our model predictions ( Fig. 3b ). Further, our model mimicked all the observations of the latter in vitro study [28] ( Supplementary Note 3 , Supplementary Figs 1–3 ), giving us confidence in its ability to accurately unravel the behaviour of the underlying network. 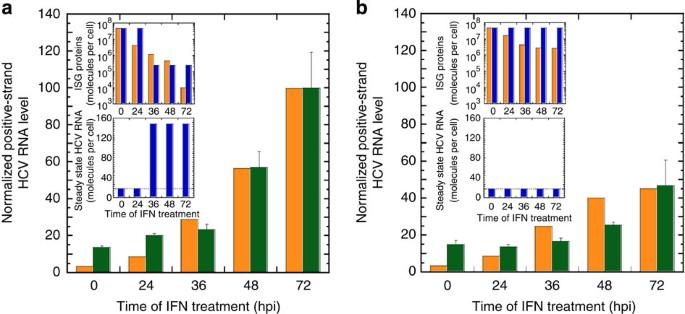Figure 3: Model validation againstin vitrodata. Normalized positive-strand HCV RNA levels predicted by our model (orange) and measured previously inin vitroexperiments28(green) at 20 h post IFN treatment (100 IU ml−1) following different specified times (hours post infection) with HCV. Error bars represent standard deviations from triplicates. Lower inset: model predictions of corresponding HCV RNA levels achieved at steady state post IFN treatment. Upper inset: model predictions of corresponding ISG protein levels at 20 h (orange) and at steady state (blue) post IFN treatment. (a) normal cells and (b), PKR-silenced cells (60% reduction in PKR mRNA transcription rate). The dashed line marks zero. Normalization was done with the positive-strand HCV RNA level in cells without IFN treatment. Parameters employed are listed inSupplementary Tables 1–3. Figure 3: Model validation against in vitro data. Normalized positive-strand HCV RNA levels predicted by our model (orange) and measured previously in in vitro experiments [28] (green) at 20 h post IFN treatment (100 IU ml −1 ) following different specified times (hours post infection) with HCV. Error bars represent standard deviations from triplicates. Lower inset: model predictions of corresponding HCV RNA levels achieved at steady state post IFN treatment. Upper inset: model predictions of corresponding ISG protein levels at 20 h (orange) and at steady state (blue) post IFN treatment. ( a ) normal cells and ( b ), PKR-silenced cells (60% reduction in PKR mRNA transcription rate). The dashed line marks zero. Normalization was done with the positive-strand HCV RNA level in cells without IFN treatment. Parameters employed are listed in Supplementary Tables 1–3 . Full size image Diversity of the cellular response to IFN We found that the network exhibited bistability over several-fold changes in the values of several parameters ( Supplementary Fig. 4 ). Global sensitivity analysis yielded parameters to which the systems-level properties of the network were sensitive ( Supplementary Note 4 , Supplementary Fig. 4 ). Bistability was lost when parameter values tilted the competition between HCV and IFN heavily in favour of either one. For instance, when the repression coefficients for the control of HCV replication by ISGs were decreased, IFN effectiveness increased and the system admitted the steady state Q 3 alone, where HCV is eliminated. When the repression coefficients were increased, IFN effectiveness decreased and the system admitted Q 1 alone, where HCV thrives ( Fig. 4a ). 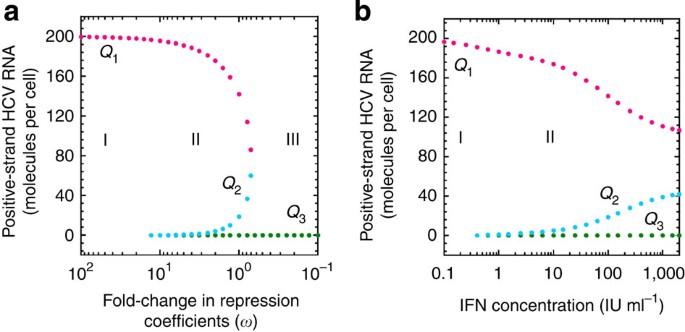Figure 4: Hysteresis and distinct cellular responses to IFN. Steady states of the network,Q1(pink),Q2(cyan) andQ3(green) over a range of values of (a), the repression coefficients for the control of HCV replication by ISGs (ωdenotes the fold-change in the repression coefficients of all ISGs relative to their baseline values inSupplementary Table 3), and (b), the IFN level. The three distinct cellular response phenotypes (see text) are marked. Region I admitsQ1alone, region II bothQ1andQ3and region IIIQ3alone. Inb, region III does not occur within the range of IFN levels considered. Other parameters employed are listed inSupplementary Tables 1–3. Figure 4: Hysteresis and distinct cellular responses to IFN. Steady states of the network, Q 1 (pink), Q 2 (cyan) and Q 3 (green) over a range of values of ( a ), the repression coefficients for the control of HCV replication by ISGs ( ω denotes the fold-change in the repression coefficients of all ISGs relative to their baseline values in Supplementary Table 3 ), and ( b ), the IFN level. The three distinct cellular response phenotypes (see text) are marked. Region I admits Q 1 alone, region II both Q 1 and Q 3 and region III Q 3 alone. In b , region III does not occur within the range of IFN levels considered. Other parameters employed are listed in Supplementary Tables 1–3 . Full size image It follows that intrinsic variations across cells, for example, in ISG expression [44] , [45] or the expression of host protease and other enzymes that affect HCV replication, would yield three distinct cellular phenotypes based on the response to a given level of IFN stimulation, viz., cells that admit Q 1 alone, Q 3 alone or both Q 1 and Q 3 . Cells that admit Q 1 alone would allow HCV persistence even with IFN stimulation. Cells that admit Q 3 alone would clear HCV following IFN stimulation. Cells that admit both Q 1 and Q 3 would either allow HCV persistence or clear HCV depending on the time of IFN addition, as illustrated above. Increasing the level of IFN stimulation could convert a cell that admits Q 1 alone to one that admits both Q 1 and Q 3 and further to one that admits Q 3 alone. Decreasing the level of IFN stimulation could reverse these transitions. Bistable systems, however, display hysteretic behaviour: the level of IFN stimulation required to drive a cell from Q 1 to Q 3 would be larger than the level at which the cell transitions from Q 3 to Q 1 . The former level may lie beyond experimentally/clinically employed levels of IFN [28] ( Fig. 4b ). Thus, cells in the state Q 1 may allow HCV persistence despite seemingly high levels of IFN stimulation and are therefore predicted to be refractory to IFN. In contrast, cells in the state Q 3 clear HCV infection with much lower levels of IFN stimulation following exposure to HCV ( Fig. 4b ). The latter cells are thus sensitive to IFN. How an HCV-infected individual responds to IFN-based treatment would thus be determined by the distribution of cells in the individual across the different IFN response phenotypes. Viral kinetics and treatment outcome To predict the ensuing viral kinetics and treatment outcome, we advanced the basic model of viral kinetics in vivo [14] , [46] , [47] , [48] , [49] ( Supplementary Note 5 ) by explicitly considering cell subpopulations with the three distinct IFN response phenotypes ( Fig. 5a ). We divided target cells into subpopulations T i with i =1, 2 and 3 representing cells that admit Q 1 alone, both Q 1 and Q 3 , and Q 3 alone, respectively, at the level of IFN exposure employed in the treatment; because ribavirin potentiates IFN activity, the subpopulations may be defined based on the combined activity of PR. Correspondingly, infected cells are divided into subpopulations I 1 , I 2 and I 3 . From the above analysis, it follows that cells T 1 remain susceptible to infection and are refractory to IFN. IFN does not inhibit de novo infection in this subpopulation. Cells T 2 are sensitive to IFN, as IFN exposure before HCV infection drives these cells to the state Q 3 and prevents de novo infections. Cells T 3 are similarly protected from new infections. Cells I 1 are again refractory to IFN and continue viral production. Cells I 2 are infected before IFN exposure and thus attain the state Q 1 following IFN exposure and continue to produce virions. Cells I 3 admit Q 3 alone and are cured following exposure to IFN. 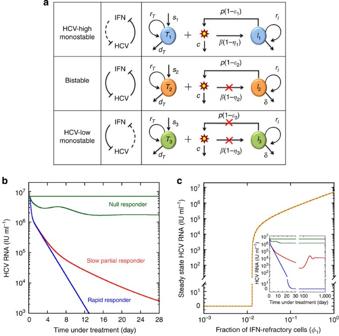Figure 5: Viral kinetics following IFN treatment. (a) Schematic of viral kinetics incorporating distinct cellular responses to IFN. Top: cells that have poor IFN control of HCV (left) admitQ1alone and are refractory to IFN (right). Middle: cells that have intermediate IFN control of HCV and vice versa (left) admit bothQ1andQ3and thus continue viral production when infected but are protected from new infections by IFN (right). Bottom: cells that have strong IFN control of HCV (left) admitQ3alone and are sensitive to IFN (right). Target cells in the three subpopulations,Ti, wherei=1, 2 and 3, are produced at the ratessi, proliferate with the rate constantrT, die with the rate constantdTand are lost owing tode novoinfection with the rate constantβ. The corresponding infected cellsIiproliferate with the rate constantrIand die with the rate constantδ. Free virions are produced by infected cells with the rate constantpand are cleared with the rate constantc. Thede novoinfection rate and virion production rate were assumed to be blocked with efficaciesηiandεiin the respective subpopulations owing to PR treatment. (b) Model predictions of different viral response patterns following IFN treatment for different distributions of cells in the three IFN response phenotypes:φ1=1,φ2=0, andφ3=0 (green top);φ1=0.35,φ2=0.35, andφ3=0.3 (green bottom);φ1=0.015,φ2=0.185, andφ3=0.8 (red); andφ1=0,φ2=0.2, andφ3=0.8 (blue). (c) Steady state viral levels following IFN treatment as a function ofφ1whenφ2=φ3(solid line) andφ2=0.5φ3(dashed line) (the two curves overlap) and (Inset) long-term virological response corresponding to the predictions inb. Parameters:V0=7 × 106IU ml−1,β=3 × 10−7ml per virions per day. Other parameter values employed are listed inSupplementary Table 4. Figure 5: Viral kinetics following IFN treatment. ( a ) Schematic of viral kinetics incorporating distinct cellular responses to IFN. Top: cells that have poor IFN control of HCV (left) admit Q 1 alone and are refractory to IFN (right). Middle: cells that have intermediate IFN control of HCV and vice versa (left) admit both Q 1 and Q 3 and thus continue viral production when infected but are protected from new infections by IFN (right). Bottom: cells that have strong IFN control of HCV (left) admit Q 3 alone and are sensitive to IFN (right). Target cells in the three subpopulations, T i , where i =1, 2 and 3, are produced at the rates s i , proliferate with the rate constant r T , die with the rate constant d T and are lost owing to de novo infection with the rate constant β . The corresponding infected cells I i proliferate with the rate constant r I and die with the rate constant δ . Free virions are produced by infected cells with the rate constant p and are cleared with the rate constant c . The de novo infection rate and virion production rate were assumed to be blocked with efficacies η i and ε i in the respective subpopulations owing to PR treatment. ( b ) Model predictions of different viral response patterns following IFN treatment for different distributions of cells in the three IFN response phenotypes: φ 1 =1, φ 2 =0, and φ 3 =0 (green top); φ 1 =0.35, φ 2 =0.35, and φ 3 =0.3 (green bottom); φ 1 =0.015, φ 2 =0.185, and φ 3 =0.8 (red); and φ 1 =0, φ 2 =0.2, and φ 3 =0.8 (blue). ( c ) Steady state viral levels following IFN treatment as a function of φ 1 when φ 2 = φ 3 (solid line) and φ 2 =0.5 φ 3 (dashed line) (the two curves overlap) and (Inset) long-term virological response corresponding to the predictions in b . Parameters: V 0 =7 × 10 6 IU ml −1 , β =3 × 10 −7 ml per virions per day. Other parameter values employed are listed in Supplementary Table 4 . Full size image The resulting viral kinetics typically follows a biphasic decline ( Fig. 5b ). We estimate with our model that the viral load at the end of the first phase is ~ V 0 (1– φ 3 ), where V 0 is the baseline viral load and φ 3 is the pre-treatment frequency of IFN-sensitive cells ( Supplementary Note 6 , Supplementary Fig. 5A ). The extent of the first phase decline is thus determined by the fraction of cells cured by IFN. The second phase slope depends on the dynamics of the infected cells. Whereas cells I 2 and I 3 decline at the death rate δ — de novo infection is blocked by IFN in these subpopulations and infected cells are expected not to proliferate significantly [48] ( Supplementary Table 4 )—the loss of cells I 1 is compensated at least in part by the de novo infection of cells T 1 , refractory to IFN ( Supplementary Note 5 , Supplementary Fig. 5B ). The early second phase slope estimated using our model is ~ δ (1– φ 1 ). The second phase slope thus decreases as the pre-treatment frequency of IFN-refractory cells, φ 1 , increases ( Supplementary Note 6 , Supplementary Fig. 5C ). By varying the frequencies φ 1 , φ 2 and φ 3 , our model reproduced all the patterns of viral kinetics observed in patients ( Fig. 5b ). The second phase slope in our model depends on φ 1 . Indeed, we find that when φ 1 is below a critical value, , viral clearance is achieved ( Fig. 5c ). This critical value does not depend on φ 2 and φ 3 because following treatment, cells T 2 and T 3 do not acquire new infections and cells I 2 and I 3 are eventually lost owing to cell death even when IFN fails to cure them. IFN-refractory cells, T 1 , remain susceptible to new infections even during treatment and thus determine treatment outcome. When their number is sufficiently small, viral production from infected cells is inadequate to replenish the loss of infected cells owing to cell death (akin to the basic reproductive number being below unity [50] ), resulting in the eventual clearance of infection. Thus, the success of IFN treatment depends primarily on the size of the IFN-refractory subpopulation. The larger the latter subpopulation, the smaller the second phase slope, thus presenting an explanation of the strong correlation observed between the second phase slope and treatment response [46] , [51] , [52] . Comparison with patient data We next applied our model to analyze data of viral kinetics obtained previously from patients under IFN monotherapy [46] . Our model provided excellent fits to the data ( Fig. 6a , Supplementary Fig. 6 , Supplementary Tables 5 and 6 ). In agreement with our prediction above, we found from the fits that , an upper bound on φ 1 obtained by letting φ 2 =0, increased from 0.01 for a typical rapid responder, to 0.11 for a slow partial responder and 0.37 for a null responder. Similarly, patients with known favourable haplotypes based on SNPs in the IFN-λ locus had significantly lower on an average than patients with unfavourable haplotypes ( Supplementary Fig. 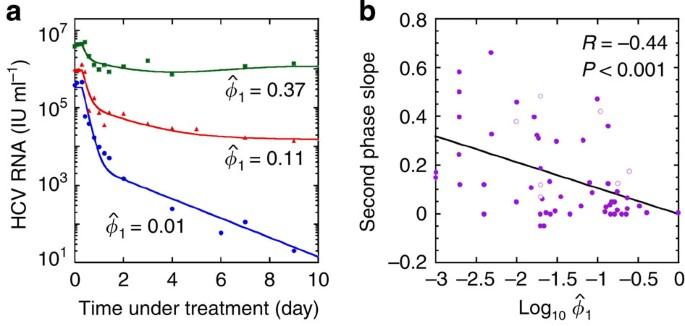Figure 6: Analysis of patient data. (a) Fits of model predictions of viral load decay following IFN treatment (lines) to previous patient data46(symbols), where the decay patterns mimic typical null responders (green), slow partial responders (red) and rapid responders (blue). We fixed known model parameter values from the literature46,48,49(Supplementary Table 4). We let inter-patient variations be determined by the parametersβandV0and the distribution of cells in the three IFN response phenotypes,φ1,φ2andφ3. We recognized thatφ3is determined by the viral load decline in the first phase (see text). The available second phase data did not allow the estimation of bothφ1andφ2uniquely. We therefore assumedφ2=0 and estimatedas the corresponding upper bound onφ1. We thus letβ,V0andbe adjustable parameters. The resulting estimates of, which were robust to variations in the fixed parameters (Supplementary Fig. 11), are mentioned above. The best-fit parameter estimates and measures of goodness of fit are listed inSupplementary Table 5. Other parameter values employed are listed inSupplementary Table 4. (b) Pre-treatment frequency of IFN-refractory cells and the slope of the second phase decline estimated from data in two reports on patients under IFN monotherapy (closed circles: ref.51; open circles: ref.53) are strongly correlated (Pearson’s correlation coefficient,R=−0.44,P<0.001). Using the standard model of viral dynamics, the efficacy of IFN,ε, and the death rate of infected cells,δ, were estimated from previously published data of viral kinetics for the patients51,53. The second phase slope is the productδεaccording to the standard model. Further,εin the standard model corresponds toφ3in our model, which yielded. 6 , Supplementary Table 6 ). Finally, we estimated for a large set of patients under IFN monotherapy [51] , [53] and found it to be negatively correlated with the second phase slope ( Fig. 6b ), reiterating the dependence of the second phase slope and hence treatment outcome on the frequency of IFN-refractory cells. Figure 6: Analysis of patient data. ( a ) Fits of model predictions of viral load decay following IFN treatment (lines) to previous patient data [46] (symbols), where the decay patterns mimic typical null responders (green), slow partial responders (red) and rapid responders (blue). We fixed known model parameter values from the literature [46] , [48] , [49] ( Supplementary Table 4 ). We let inter-patient variations be determined by the parameters β and V 0 and the distribution of cells in the three IFN response phenotypes, φ 1 , φ 2 and φ 3 . We recognized that φ 3 is determined by the viral load decline in the first phase (see text). The available second phase data did not allow the estimation of both φ 1 and φ 2 uniquely. We therefore assumed φ 2 =0 and estimated as the corresponding upper bound on φ 1 . We thus let β , V 0 and be adjustable parameters. The resulting estimates of , which were robust to variations in the fixed parameters ( Supplementary Fig. 11 ), are mentioned above. The best-fit parameter estimates and measures of goodness of fit are listed in Supplementary Table 5 . Other parameter values employed are listed in Supplementary Table 4 . ( b ) Pre-treatment frequency of IFN-refractory cells and the slope of the second phase decline estimated from data in two reports on patients under IFN monotherapy (closed circles: ref. 51 ; open circles: ref. 53 ) are strongly correlated (Pearson’s correlation coefficient, R =−0.44, P <0.001). Using the standard model of viral dynamics, the efficacy of IFN, ε , and the death rate of infected cells, δ , were estimated from previously published data of viral kinetics for the patients [51] , [53] . The second phase slope is the product δε according to the standard model. Further, ε in the standard model corresponds to φ 3 in our model, which yielded . Full size image Pre- and post-treatment ISG expression and response to IFN We next examined how treatment response correlated with pre- and post-treatment ISG expression. The pre-treatment frequency of cells refractory to IFN would depend on the level of endogenous IFN production following infection as well as the strength of the effector function of ISGs, or, more generally, the effector function of the IFN network. IFN production stimulates the IFN network, whose effector function determines the propensity to clear HCV. Four possibilities thus arise ( Fig. 7 ). 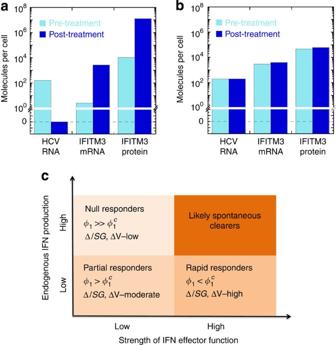Figure 7: Pre- and post-treatment ISG expression and treatment response. Pre- and post-treatment steady state positive-strand HCV RNA, ISG mRNA and ISG protein expression levels, in (a), an IFN-sensitive cell with low endogenous IFN level (IFNendo=0.05 U ml−1) and potent IFN effector function (ω=0.5,γ=1), representative of responders, and (b), an IFN-refractory cell with high-endogenous IFN level (IFNendo=100 U ml−1) but poor effector function (ω=20,γ=0.1), representative of nonresponders. The dashed line marks zero. IFITM3 is shown as a representative ISG; other ISGs behave similarly. (c) Schematic of expected responses to IFN-based treatment in patients with different endogenous IFN production levels and potencies of IFN effector function.φ1is the pre-treatment frequency of IFN-refractory cells,is the critical pre-treatment frequency of IFN-refractory cells for successful treatment response, ΔVis the fold-decline in viral load and ΔISGis the fold increase in ISG mRNA levels relative to their respective pre-treatment levels.ωandγrepresent the fold changes in the repression coefficients of all ISGs and the eIF2B production rate constant, respectively, relative to their baseline values inSupplementary Table 3. Parameters:IFNexo=100 U ml−1. Other parameters are listed inSupplementary Tables 1–3. Figure 7: Pre- and post-treatment ISG expression and treatment response. Pre- and post-treatment steady state positive-strand HCV RNA, ISG mRNA and ISG protein expression levels, in ( a ), an IFN-sensitive cell with low endogenous IFN level ( IFN endo =0.05 U ml −1 ) and potent IFN effector function ( ω =0.5, γ =1), representative of responders, and ( b ), an IFN-refractory cell with high-endogenous IFN level ( IFN endo =100 U ml −1 ) but poor effector function ( ω =20, γ =0.1), representative of nonresponders. The dashed line marks zero. IFITM3 is shown as a representative ISG; other ISGs behave similarly. ( c ) Schematic of expected responses to IFN-based treatment in patients with different endogenous IFN production levels and potencies of IFN effector function. φ 1 is the pre-treatment frequency of IFN-refractory cells, is the critical pre-treatment frequency of IFN-refractory cells for successful treatment response, Δ V is the fold-decline in viral load and Δ ISG is the fold increase in ISG mRNA levels relative to their respective pre-treatment levels. ω and γ represent the fold changes in the repression coefficients of all ISGs and the eIF2B production rate constant, respectively, relative to their baseline values in Supplementary Table 3 . Parameters: IFN exo =100 U ml −1 . Other parameters are listed in Supplementary Tables 1–3 . Full size image When endogenous IFN production is low (for example, owing to HCV-mediated cleavage of mitochondrial antiviral signaling protein (MAVS) [43] , [54] ) and IFN effector function potent, infection is established because of inadequate stimulation of the IFN network. ISG levels are predicted to be low in such individuals before treatment ( Fig. 7a ). Exogenous IFN addition during treatment stimulates the IFN network, which increases ISG expression and, given potent IFN effector function, clears infection. Cells in such individuals predominantly admit Q 3 at the level of IFN exposure during treatment. Such individuals are predicted to be rapid responders to IFN treatment ( Fig. 7c ). When endogenous IFN production is high but IFN effector function compromised, infection is established despite stimulation of the IFN network. Here ISG levels are high before treatment ( Fig. 7b ), but HCV continues to thrive because of poor effector function. Cells in such individuals predominantly admit Q 1 and addition of exogenous IFN contributes little to the control of infection. Such individuals are predicted to be null responders to treatment ( Fig. 7c ). When both endogenous IFN production and ISG effectiveness are low, addition of IFN may increase ISG levels but not necessarily clear HCV given the inadequate effector function. Such individuals appear as partial responders. The fraction of IFN-refractory cells is smaller in such individuals than in null responders, but treatment would fail as long as the fraction is larger than the critical value mentioned above. When both endogenous IFN production and ISG effectiveness are high, infection is likely to be spontaneously cleared; spontaneous clearance has been observed to additionally require strong cytotoxic T-cell responses [22] , which our study did not consider. We note that IFN effector function is compromised at steps downstream of the step(s) in the IFN signalling network at which HCV interferes. For instance, HCV interfered above at the level of ISG translation, so that poor effector function arose from low levels of ISG proteins despite high-ISG mRNA levels. In this case, both uninfected and infected cells would display high-pre-treatment ISG mRNA expression in nonresponders. If, instead, HCV were to predominantly inhibit the JAK–STAT pathway, low effector function would arise from low ISG mRNA expression. High-pre-treatment ISG expression in nonresponders would then be restricted to uninfected cells via paracrine signalling. Synergy between DAAs and IFN Finally, we examined the origin of the synergy between DAAs and IFN. DAAs such as HCV protease and polymerase inhibitors lower the HCV replication rate and would therefore weaken the control of HCV on the IFN network. To characterize the impact of such a DAA, we identified the steady states of the network at different (dose-dependent) DAA efficacies ( Fig. 8a ). At low DAA efficacies, the system again exhibits the bistable behaviour observed earlier. As the efficacy increases, the HCV RNA level corresponding to Q 1 declines and that corresponding to Q 2 increases. Interestingly, beyond a critical efficacy, the HCV-high state is rendered unsustainable and the system jumps to Q 3 where HCV is cleared. The DAA thus transforms a bistable cell into a cell that admits Q 3 alone. Similarly, a cell that admits Q 1 alone could be transformed into one that admits both Q 1 and Q 3 ( Fig. 8b ). At the cell population level, this effect of the DAA would manifest as an increase in the fraction of IFN-sensitive cells, φ 3 , at the expense of IFN-refractory cells, φ 1 , and thus result in improved treatment response. 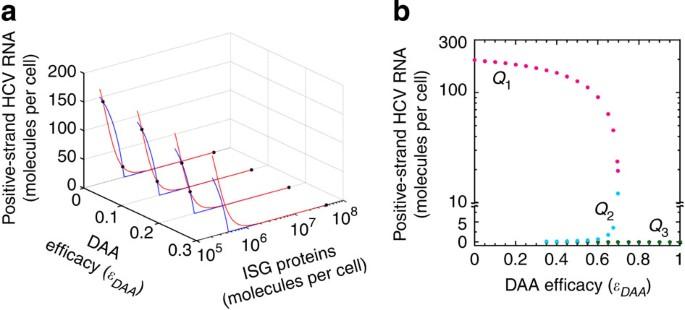Figure 8: Influence of DAA on IFN responsiveness. (a) Concentration-effect curves showing steady state positive-strand HCV RNA levels for fixed ISG protein levels (blue lines) and ISG protein levels for fixed double-stranded HCV RNA levels (red lines) in the presence of a DAA at different efficacies (εDAA). (b) Steady states of the network as a function of DAA efficacy. Ina,ω=1,γ=1. Inb,ω=10,γ=0.1.ωandγrepresent the fold changes in the repression coefficients of all ISGs and the eIF2B production rate constant, respectively, relative to their baseline values inSupplementary Table 3. Other parameters are listed inSupplementary Tables 1–3. Figure 8: Influence of DAA on IFN responsiveness. ( a ) Concentration-effect curves showing steady state positive-strand HCV RNA levels for fixed ISG protein levels (blue lines) and ISG protein levels for fixed double-stranded HCV RNA levels (red lines) in the presence of a DAA at different efficacies ( ε DAA ). ( b ) Steady states of the network as a function of DAA efficacy. In a , ω =1, γ =1. In b , ω =10, γ =0.1. ω and γ represent the fold changes in the repression coefficients of all ISGs and the eIF2B production rate constant, respectively, relative to their baseline values in Supplementary Table 3 . Other parameters are listed in Supplementary Tables 1–3 . Full size image A hallmark of HCV infection has been its persistence in many individuals despite strong ISG expression in the liver and high doses of IFN and ribavirin [8] , [9] , [10] . What underlies this persistence has remained poorly understood. In the present study, we provide a new conceptual basis for understanding HCV persistence and response to IFN-based treatment. Negative regulators of the IFN system, such as SOCS and USP18, as well as the recently identified IFN-associated immunosuppression have been suggested to contribute to viral persistence despite IFN stimulation [6] , [20] , [21] . While these mechanisms are undoubtedly important, they remain partial determinants of HCV persistence and treatment response because they do not explain when pre-treatment ISG expression would be high. Further, a direct role of HCV in suppressing IFN effector function may be important in determining treatment response because DAAs that suppress HCV replication can induce SVRs in previous null responders to PR. Our study predicts that these additional mechanisms, potentially central to HCV persistence and treatment response, may arise from the systems-level properties of the IFN signalling network modulated by HCV. Our model of the IFN signalling network predicts that HCV induces bistability in the network. IFN signalling is designed to clear viral infections. HCV interferes with IFN signalling and introduces an alternative steady state where HCV persists. To our knowledge, this is the first instance identified where a virus induces bistability in an innate immune signalling network to achieve persistence. A consequence is that IFN effector function can be compromised despite high-IFN production, allowing viral persistence in the presence of high-ISG expression. Addition of exogenous IFN yields no additional antiviral effect. When more than a critical fraction of cells in an individual is refractory to IFN, treatment would fail. DAAs improve treatment response by suppressing HCV replication, which compromises the ability of HCV to induce bistability in the network, thereby lowering the fraction of cells refractory to IFN. The IFN signalling network comprises a large number of molecular components that interact via multiple feedback loops [5] . HCV interferes with the network at several levels [6] , [22] . A complex combination of molecular players as well as parameter values determining the strengths of their interactions may thus underlie the phenotypic response of an HCV-infected cell to IFN. Currently, the limited knowledge of cell-to-cell and inter-patient variations in parameter values (for example, see ref. 55 ) precludes a priori estimation of the prevalence of IFN-refractory cells in patients and hence the establishment of a quantitative link between network properties and viral kinetics. Nonetheless, we found that HCV-induced bistability is a robust emergent property of the network: in addition to the translational block induced by HCV considered above, with which current in vivo data [29] seems consistent, we examined other known modes of HCV interference of the IFN network and also negative regulation of IFN stimulation by ISG proteins. We found bistability in all cases ( Supplementary Notes 7 and 8 , Supplementary Figs 7 and 8 ). Bistability was also maintained under parameter regimes that mimicked the dynamic oscillations in HCV-induced translational inhibition observed recently [56] , [57] ( Supplementary Note 9 , Supplementary Fig. 9 ). Further, our prediction that the pre-treatment prevalence of IFN-refractory cells beyond a critical fraction leads to treatment failure is independent of the origin of the bistability. Previous models of viral kinetics have estimated the effectiveness of PR by comparisons of model predictions with viral load decline in patients [14] , [46] , [47] , [48] , [49] , [58] . Our model reproduced all the patterns of viral kinetics observed in patients by varying the fractions of cells refractory and sensitive to IFN. Alternative interpretations thus emerge of the effectiveness estimated by previous models. The extent of first phase decline, which is taken as a measure of IFN effectiveness in lowering viral production, is in our model a measure of the pre-treatment fraction of infected cells that are subsequently cured by PR. The slope of the second phase, which is taken as a combination of PR effectiveness and the loss rate of infected cells, is in our model a combination of the loss rate of infected cells and the fraction of cells refractory to PR. Larger the latter fraction, smaller the slope, and hence poorer the treatment response. The critical effectiveness of PR predicted by previous models [47] for successful treatment translates to the level of PR activity necessary to render the fraction of cells refractory to PR below the critical value identified by our model. Our model thus presents an alternative yet equally consistent description of viral kinetics and one that is rooted in the properties of the IFN network. The synergy between DAAs and IFN predicted by our model can be compromised by the emergence of resistance to DAAs, which we did not consider. Recent studies have reported the dependence of viral kinetics on SNPs even in IFN-free treatment regimens [59] , [60] and recent trials with some two-DAA combinations without PR have been stunningly successful with >90% SVR in previous null responders to PR [61] . We speculate that this success may arise from a combination of three modes of DAA action. First, the DAAs may directly suppress HCV replication. Second, they may render cells monostable and facilitate HCV clearance. Third, the resulting lower HCV levels may lead to lower IFN stimulation, which in the absence of exogenous IFN may undo the immunosuppression caused by persistent IFN signalling and effect a cure. Identifying which of these mechanisms predominates in vivo awaits new investigations and may inform future strategies of intervention. Mathematical model of the IFN signalling network We modelled the network ( Fig. 1 ) based on mass action and Michaelis–Menten kinetics ( Supplementary Note 1 ). The parameters involved ( Supplementary Tables 1–3 ) were either obtained from the literature or estimated from analysis of independent experiments of intracellular HCV RNA kinetics ( Supplementary Figs 3 and 10 ), ISG expression following stimulation with IFN, and suppression of HCV RNA by over-expression of ISGs ( Supplementary Note 2 ). The fit of this model to the highly infectious HCV JFH-m4 strain can be found in Supplementary Fig. 10 and Supplementary Note 2 . Mathematical model of viral kinetics We modified the standard model of HCV viral kinetics to incorporate subpopulations of cells with distinct phenotypic responses to IFN ( Fig. 4 , Supplementary Note 5 ). We obtained analytical approximations to the resulting first and early second phase slopes ( Supplementary Note 6 ). The parameter values employed were obtained from the literature or estimated from fits to patient data ( Supplementary Tables 4–6 ). Solution of model equations and data analysis We solved the model of the IFN signalling network and the model of viral kinetics using the Rosenbrock algorithm in Berkeley-Madonna version 8.3.18 and the ode15s routine in MATLAB. We fit the model predictions to the data using the nonlinear regression tool NLINFIT in MATLAB and estimated 95% confidence intervals using the tool NLPARCI in MATLAB. We assessed the goodness of fits using R 2 and the Student’s t -test on residuals. All data digitization was done using Engauge digitizer. The computer programs employed are available upon request. How to cite this article: Padmanabhan, P. et al. Emergent properties of the interferon-signalling network may underlie the success of hepatitis C treatment. Nat. Commun. 5:3872 doi: 10.1038/ncomms4872 (2014).